Antagonism between binding site affinity and conformational dynamics tunes alternativecis-interactions within Shp2 Protein functions are largely affected by their conformations. This is exemplified in proteins containing modular domains. However, the evolutionary dynamics that define and adapt the conformation of such modular proteins remain elusive. Here we show that cis -interactions between the C-terminal phosphotyrosines and SH2 domain within the protein tyrosine phosphatase Shp2 can be tuned by an adaptor protein, Grb2. The competitiveness of two phosphotyrosines, namely pY542 and pY580, for cis -interaction with the same SH2 domain is governed by an antagonistic combination of contextual amino acid sequence and position of the phosphotyrosines. Specifically, pY580 with the combination of a favourable position and an adverse sequence has an overall advantage over pY542. Swapping the sequences of pY542 and pY580 results in one dominant form of cis -interaction and subsequently inhibits the trans -regulation by Grb2. Thus, the antagonistic combination of sequence and position may serve as a basic design principle for proteins with tunable conformations. Intramolecular interactions within proteins ( cis -interactions) and allosteric regulations by neighbouring molecules ( trans -interactions) are common ways to regulate protein functions. One mode of cis -interaction is autoinhibition in which a cis -regulatory element interacts with and inhibits the catalytic/functional domain. Disruption of the cis -interaction usually involves a neighbouring molecule trans -interacting with the cis -regulatory element and relieving the autoinhibition to activate the protein [1] . In these interactions, modularity is a recurring theme to regulate diverse functions of proteins [2] . While the specific sequence and position of DNA cis -regulatory elements have been intensively studied to elucidate their roles in regulating gene expression [3] , [4] , [5] , the basic principles underlying how protein modules are designed and arranged to govern their conformations and functions remain largely elusive. X-ray crystallography, NMR spectroscopy and single-molecule spectroscopic methods can provide details of molecular conformations in vitro , but have limited capability in live cells, particularly for proteins containing multiple interacting domains and capable of adopting diverse conformations [6] . Genetically encoded reporters based on fluorescent proteins (FPs) and fluorescence resonance energy transfer (FRET) allow the monitoring of the molecular interactions and conformational changes in live cells with high spatiotemporal resolution [7] , [8] , [9] , [10] . In this study, we employed FRET to study the cis - and trans -interactions of Src homology 2 domain-containing protein tyrosine phosphatase 2 (Shp2). Encoded by PTPN11 , Shp2 is a protein tyrosine phosphatase (PTP) that has a critical role in various pathophysiological processes [11] , [12] , [13] . Mutations of PTPN11 cause Noonan Syndrome [14] , LEOPARD syndrome [15] and juvenile myelomonocytic leukaemia [16] , [17] . Structurally, Shp2 consists of two Src homology 2 (SH2) domains (N-SH2 and C-SH2), a PTP domain, and a C-terminal tail (C-tail) containing two major tyrosine sites (Y542 and Y580) (ref. 18 ). By incorporating non-hydrolysable phosphonomethylene phenylalanine at either Y542 or Y580, it has been suggested that these unnatural chemical modifications mimicking phosphotyrosines may cause the coupling between intramolecular domains in vitro to alter phosphatase activity of Shp2 (ref. 19 ). However, it is unclear how the protein modules within Shp2 are designed for the cis -regulation and coordination of physiological Shp2 functions in live cells. We have developed a FRET-based reporter to visualize conformational changes of Shp2 and their underlying regulation mechanisms in live cells. Our results indicate that an antagonistic combination of contextual amino acid (aa) sequence and position of Y542 and Y580 within Shp2 facilitates the effective tuning of Shp2 cis -interactions by Grb2-mediated trans -regulation. The disruption of this antagonistic combination results in the inhibition of trans -regulation of Shp2 conformations and reprograms kinetics of the downstream extracellular signal-regulated kinase (ERK) signalling. We suggest that this antagonistic combination of sequence and position may serve as a basic design principle for proteins with tunable conformations and functions. FRET-based reporter reveals cis -interaction of Shp2 in vitro We studied the Shp2 conformations by engineering FRET reporters containing a full-length wild-type (WT) Shp2 flanked by a sensitive FRET pair, an enhanced cyan FP (ECFP) and a yellow FP variant (YFP for energy transfer (YPet)) [20] ( Fig. 1a ). The purified WT reporter in vitro can be phosphorylated by platelet-derived growth factor receptor (PDGFR)β kinase at both Y542 and Y580 ( Fig. 1b ), concomitant with an enhanced FRET level represented by an increase in YPet and a decrease in ECFP emission ( Fig. 1c ). The sustained FRET increase of the WT reporter suggests that PDGFRβ kinase activity is dominant over intrinsic phosphatase activity of the Shp2 reporter ( Fig. 1d ). Consistently, the incubation with extra amount of kinase did not cause further increase of the overall level of FRET signals ( Supplementary Fig. S1a ). In contrast, PDGFRβ caused the phosphorylation but not FRET change of a mixture containing ECFP–Shp2 (ECFP fused to Shp2) and Shp2–YPet (YPet fused to Shp2) ( Supplementary Fig. S1b ), indicating minimal intermolecular interactions ( trans -interactions) between different copies of Shp2 reporters. Furthermore, the PDGFRβ-induced FRET increase was lost in the YDF reporter with mutations of both Y542 and Y580 ( Fig. 1d ), which still has intact SH2 domains capable of trans -interaction with the phosphorylated Y1009 of PDGFRβ in the assay [21] . Therefore, the FRET response of WT reporter cannot be attributed to its interaction with PDGFRβ either, and must arise from intramolecular interactions ( cis -interactions) within Shp2. 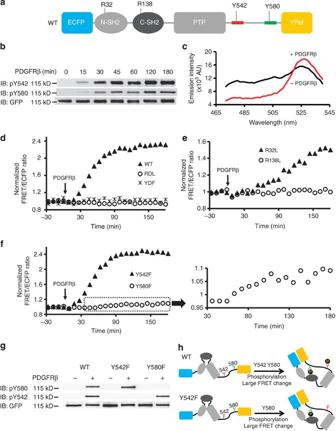Figure 1:cis-Interactions of the Shp2 reportersin vitro. (a) Schematic drawing of the WT Shp2 reporter, with mutation sites as indicated. Y542 and Y580 sequences are coloured in red and green, respectively. (b) The phosphorylation of the WT reporter upon PDGFRβ incubationin vitro(refer toSupplementary Fig. S6afor the whole blots). (c) The emission spectrum change of the WT reporter before (black) and after (red) PDGFRβ incubation. (d–f) The ratio time courses of the WT reporter and its mutants as indicated. (f) Inset shows the time course of zoom-in ratios of Y580F reporter upon PDGFRβ incubation. (g) The tyrosine phosphorylation of Y580 and Y542 of the WT reporter, its Y542F or Y580F mutantin vitrobefore and after PDGFRβ incubation. (h) The models depict thecis-interactions and FRET changes of the WT and Y542F reporters upon phosphorylationin vitro. AU, arbitrary unit. Figure 1: cis -Interactions of the Shp2 reporters in vitro . ( a ) Schematic drawing of the WT Shp2 reporter, with mutation sites as indicated. Y542 and Y580 sequences are coloured in red and green, respectively. ( b ) The phosphorylation of the WT reporter upon PDGFRβ incubation in vitro (refer to Supplementary Fig. S6a for the whole blots). ( c ) The emission spectrum change of the WT reporter before (black) and after (red) PDGFRβ incubation. ( d–f ) The ratio time courses of the WT reporter and its mutants as indicated. ( f ) Inset shows the time course of zoom-in ratios of Y580F reporter upon PDGFRβ incubation. ( g ) The tyrosine phosphorylation of Y580 and Y542 of the WT reporter, its Y542F or Y580F mutant in vitro before and after PDGFRβ incubation. ( h ) The models depict the cis -interactions and FRET changes of the WT and Y542F reporters upon phosphorylation in vitro . AU, arbitrary unit. Full size image C-SH2 dominates the cis -interaction in vitro The PDGFRβ-induced FRET response was eliminated by YDF or the double SH2 domain mutant (RDL) ( Fig. 1d ), suggesting that the cis -interactions within Shp2 are mediated by its SH2 domains and phosphotyrosines at C-tail. Single C-SH2 mutation (R138L), but not N-SH2 mutation (R32L), eliminated the PDGFRβ-induced FRET increase ( Fig. 1e ), indicating that C-SH2 is essential for the cis -interaction. Y580F, but not Y542F mutation, blocked most FRET increase ( Fig. 1f ), even though the phosphorylation of these two mutants was similar to that of WT reporters ( Fig. 1g ). Therefore, the FRET response of WT reporter in vitro is mainly due to the cis -interaction between C-SH2 and phosphorylated Y580 (pY580) ( Fig. 1h ). This notion is further supported by the obvious FRET response of a mutant disrupting the functions of both N-SH2 and Y542 (R32LY542F) ( Supplementary Fig. S1c ). cis -Interaction competitiveness of the phosphotyrosines Interestingly, there was a consistent although minor FRET response of the Y580F reporter ( Fig. 1f and inset), suggesting that phosphorylated Y542 (pY542) may also undergo cis -interaction with C-SH2 in the absence of pY580 but only yield a weak FRET change. The reason for this weak FRET may come from the 51aa-long flexible C-tail region of the Y580F reporter between pY542 (the C-SH2-binding site) and YPet (the FRET acceptor) ( Fig. 2a ), in contrast to the short 13aa-region between pY580 and YPet in WT and Y542F reporters ( Fig. 1h ). Indeed, truncating this 51aa-long region (Δ580) to 13aa ( Fig. 2a ) caused a substantial FRET increase upon PDGFRβ incubation ( Fig. 2b ), which can be abolished by additional C-SH2 (R138L) but not N-SH2 (R32L) mutation ( Supplementary Fig. S1d ). These results confirmed that the cis -interaction between pY542 and C-SH2 can occur in the absence of pY580 ( Fig. 2a ). However, pY580 dominates the cis -interactions with C-SH2 in the population of WT reporters because the conversion of weak-FRET population, if any, to high FRET by Y542F mutation did not cause any significant increase in the overall FRET response ( Fig. 1d ). As both tyrosine sites are phosphorylated in the WT reporter ( Fig. 1g ), we suspect that the aa sequence surrounding pY580 has a higher affinity binding to C-SH2. Surprisingly, direct affinity measurement of the isolated pY542 or pY580 peptide towards C-SH2 by surface plasmon resonance (SPR) revealed a much higher binding affinity between pY542 and C-SH2 ( Fig. 2c and Table 1 ). Furthermore, when the Y542 sequence was truncated so that it was replaced by the relocated Y580 sequence (Δ542, Fig. 2a ), no FRET response was observed ( Fig. 2b ), although substantial phosphorylation of Y580 occurred ( Supplementary Fig. S1e ). As the only difference between Δ580 and Δ542 reporters is their distinct sequences at position 542 ( Fig. 2a ), the stronger FRET response of Δ580 reporter with pY542 sequence confirms that C-SH2 also favours the pY542 sequence over pY580 in the context of the whole Shp2 protein. The dominant cis -interaction between pY580 and C-SH2 within the WT reporter where both Y542 and Y580 are phosphorylated, therefore, suggests that position 580 may be favoured over position 542 for C-SH2 interaction to overpower the advantageous pY542 sequence. Indeed, when the reporter was reengineered to have identical Y542 sequence at both 542 and 580 positions (Y542Y542), position 580 is the preferred cis -interaction site for C-SH2 because a mutation at position 580 but not 542 suppressed the majority of FRET response ( Fig. 2d ). Therefore, the dominant cis -interaction between C-SH2 and pY580 within the WT reporter in vitro is resulted from an antagonistic combination of an adverse sequence but a favourable position at pY580. 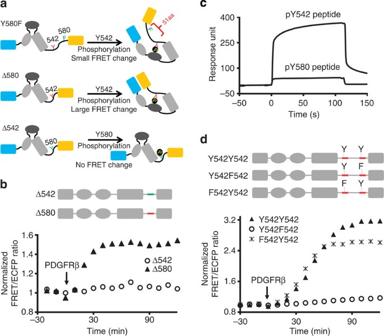Figure 2: The combination of contextual sequence and position determines the preference of phosphotyrosines forcis-interaction. (a) The models depict thecis-interactions of the Y580F, Δ580 and Δ542 reporters upon phosphorylationin vitro. (b) The ratio time courses of Δ542 and Δ580 reporters. Y542 and Y580 sequences are coloured in red and green, respectively. (c) The binding curves of the C-SH2 domain (4.5 μM) towards immobilized pY542 or pY580 peptides measured by SPR (refer toSupplementary Fig. S8for the binding kinetics and original sensorgrams). (d) The ratio time courses of engineered Y542Y542 and its mutant reporters as indicated. Figure 2: The combination of contextual sequence and position determines the preference of phosphotyrosines for cis -interaction. ( a ) The models depict the cis -interactions of the Y580F, Δ580 and Δ542 reporters upon phosphorylation in vitro . ( b ) The ratio time courses of Δ542 and Δ580 reporters. Y542 and Y580 sequences are coloured in red and green, respectively. ( c ) The binding curves of the C-SH2 domain (4.5 μM) towards immobilized pY542 or pY580 peptides measured by SPR (refer to Supplementary Fig. S8 for the binding kinetics and original sensorgrams). ( d ) The ratio time courses of engineered Y542Y542 and its mutant reporters as indicated. Full size image Table 1 The dissociation constant ( K d ) of different peptides towards the binding of Grb2 or C-SH2 domain of Shp2. Full size table Different conformational regulation of Shp2 in cells Both purified WT reporter and full-length Shp2 in vitro showed an increased phosphatase activity upon incubation with PDGFRβ, which can interact with the N-SH2 domain and, therefore, unmask the phosphatase domain to activate Shp2 ( Supplementary Fig. S2a ). When expressed in mouse embryonic fibroblasts (MEFs), the WT reporter was recruited to membrane ruffles after platelet-derived growth factor (PDGF) stimulation with similar localization and C-tail phosphorylation as the endogenous Shp2 ( Supplementary Fig. S2b,c ). Therefore, the Shp2 reporter has the same functional activation mechanism and localizations as the endogenous Shp2. We hence applied the Shp2 reporter to monitor Shp2 conformation regulations in mammalian cells. We confirmed that the cellular concentration of Shp2 reporter when expressed in mammalian cells to be in the range of micromolar, which is similar to the concentration used in vitro ( Supplementary Fig. S2d ). PDGF caused a FRET increase of the WT reporter in MEFs ( Fig. 3a , Supplementary Fig. S3a , and Supplementary Movie 1 ), concomitant with phosphorylation at both Y542 and Y580 ( Supplementary Fig. S2c ). In contrast, no FRET response can be observed upon PDGF stimulation in MEFs expressing both ECFP–Shp2 and Shp2–YPet ( Supplementary Fig. S3b ), confirming the cis -interaction within WT reporter for the FRET change in live cells. Consistent with our in vitro results, RDL, YDF or R138L, but not R32L mutation, abolished the FRET response ( Fig. 3b , Supplementary Fig. S3c ). Surprisingly, in marked contrast to their effects in vitro , Y542F but not Y580F mutation, eliminated the PDGF-induced FRET response in MEFs ( Fig. 3b , Supplementary Fig. S3c , Supplementary Movies 2 and 3 ). The cis -interaction between pY542 and C-SH2 is hence dominant in MEFs, in contrast to the pY580 and C-SH2 pair in vitro . Consistently, the Y580F reporter, with its Y542 intact and phosphorylated ( Fig. 3c ), had a similar level of FRET change as that of WT reporter in MEFs ( Fig. 3b ). The Δ580 reporter also had stronger FRET responses than the WT reporter in MEFs, which was abolished by additional R138L but not R32L mutation ( Supplementary Fig. S3d ). All these results confirmed the primary cis -interaction between pY542 and C-SH2 in MEFs. 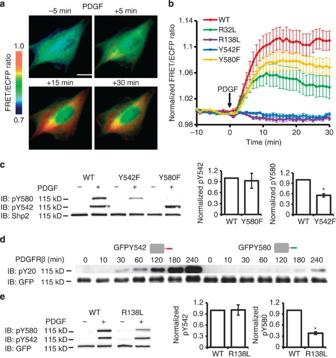Figure 3:cis-Interactions and their regulation within the Shp2 reporters in MEFs. (a) The ratiometric images of a MEF cell transfected with the WT reporter before and after PDGF stimulation for various periods of time. Scale bar, 10 mm. (b) The ratio time courses (mean±s.e.m.,n=18, 17, 15, 15 and 11) of MEFs expressing the WT reporter or its mutants. (c) The phosphorylation of WT and tyrosine mutant reporters in MEFs before and after 5 min PDGF stimulation. Bar graphs represent the mean±s.e.m. *,P<0.05. (Student’st-test,n=3, refer toSupplementary Fig. S6bfor the whole blots). (d) The tyrosine phosphorylation levels of the purified GFPY542 (1 μM) or GFPY580 (1 μM) reporter before and after 10 nM PDGFRβ incubation for indicated time periods. (e) The phosphorylation of WT and C-SH2 mutant reporters in MEFs before and after 5 min PDGF stimulation. Bar graphs represent the mean±s.e.m. *,P<0.05 (Student’st-test,n=3). Whole-cell lysate was used for panelsc,e. Figure 3: cis -Interactions and their regulation within the Shp2 reporters in MEFs. ( a ) The ratiometric images of a MEF cell transfected with the WT reporter before and after PDGF stimulation for various periods of time. Scale bar, 10 mm. ( b ) The ratio time courses (mean±s.e.m., n =18, 17, 15, 15 and 11) of MEFs expressing the WT reporter or its mutants. ( c ) The phosphorylation of WT and tyrosine mutant reporters in MEFs before and after 5 min PDGF stimulation. Bar graphs represent the mean±s.e.m. *, P <0.05. (Student’s t -test, n =3, refer to Supplementary Fig. S6b for the whole blots). ( d ) The tyrosine phosphorylation levels of the purified GFPY542 (1 μM) or GFPY580 (1 μM) reporter before and after 10 nM PDGFRβ incubation for indicated time periods. ( e ) The phosphorylation of WT and C-SH2 mutant reporters in MEFs before and after 5 min PDGF stimulation. Bar graphs represent the mean±s.e.m. *, P <0.05 (Student’s t -test, n =3). Whole-cell lysate was used for panels c,e . Full size image Y580 phosphorylation depends on Y542 and C-SH2 in MEFs We further explored the molecular mechanism underlying the distinct conformational regulations of Shp2 in vitro and in MEFs. Y580 phosphorylation in the absence of Y542 was significantly inhibited in MEFs ( Fig. 3c ) (ref. 22 ), in contrast to the independence of Y580 and Y542 phosphorylations in vitro ( Fig. 1g ). The phosphorylation of Y542 is hence essential for and may occur before Y580 phosphorylation within each copy of the reporters in MEFs. Indeed, Y542 sequence fused to green fluorescent protein (GFP) was phosphorylated substantially faster than Y580 sequence in vitro ( Fig. 3d ). R138L mutant to disrupt C-SH2 also inhibited the phosphorylation of Y580, but not that of Y542 in MEFs ( Fig. 3e ). Hence, pY542 and its subsequent cis -interaction with C-SH2 can precede and mediate the phosphorylation of Y580 in MEFs. Grb2 tunes cis -interactions and FRET levels of Shp2 reporter We then examined whether the phosphorylation of Y580, in the absence of pY542, can be rescued in MEFs to allow its cis -interaction with C-SH2 as it does in vitro . When PDGFRβ was overexpressed in MEFs, Y580 phosphorylation can occur in the absence of pY542 ( Fig. 4a ) to cause C-SH2/pY580 interaction and result in a considerable FRET change upon PDGF stimulation ( Fig. 4b ). It was puzzling then why the C-SH2/pY580 cis -interaction dominates in vitro but not in MEFs when both Y542 and Y580 are phosphorylated in the WT reporter. As the phosphorylation of Y580 follows and is dependent on the cis -interaction of C-SH2/pY542 in MEFs, we hypothesized that molecules interacting with Shp2 in MEFs, such as Grb2 (ref. 23 ), may sequester the more potent pY580 from competing for the pY542-occupied C-SH2. Indeed, purified Grb2 can reduce and tune the FRET levels when added to the phosphorylated Y542F reporter in vitro ( Fig. 4c ), by interacting with the available pY580 in the reporter ( Fig. 4d ). The amount of Grb2 can apparently cause a proportional reduction in overall FRET signals by decreasing the percentage of reporters adopting high-FRET cis -interactions ( Fig. 4c ). This tuning ability of Grb2 is mediated by its SH2 domain as the SH2-disabling mutant Grb2RV was no longer effective ( Fig. 4e ). Consistently, overexpression of Grb2 with varying concentrations can proportionally tune, via its SH2 domain, the FRET level of the Y542F reporter in MEFs overexpressing constitutively active PDGFR (Tel-PDGFRβ) [24] ( Fig. 5a ). Therefore, Grb2 can trans -interact with and sequester pY580 from cis -interaction with C-SH2 in Y542F reporter. Further results showed that Grb2 can also tune the FRET signals of WT reporter in MEFs ( Fig. 5c ). However, it is unclear whether Grb2 preferentially trans -interacts with pY580 when both Y542 and Y580 are intact and phosphorylated in the WT reporter. SPR results revealed that Grb2 has a significantly higher affinity binding to the isolated pY580 peptide than to the pY542 peptide ( Table 1 ). In addition, R138L mutation disrupting the C-SH2 occupation of pY542 in the Y580F reporter significantly increased the pY542–Grb2 interaction ( Fig. 5d ), suggesting that the preformed cis -interaction of C-SH2 and pY542 can reduce the availability of pY542 for Grb2 and hence promote Grb2–pY580 interaction in the WT reporter. Indeed, pY542 in the Y580F reporter allowed much less Grb2 binding comparing with the WT reporter ( Fig. 5e ), confirming that pY580 in Shp2 is the preferred and primary trans -interaction site for Grb2. This Grb2–pY580 association can sequester the free pY580 from competing for the pY542-occupied C-SH2, which should in turn stabilize the pY542/C-SH2 complex in MEFs ( Fig. 5f ). 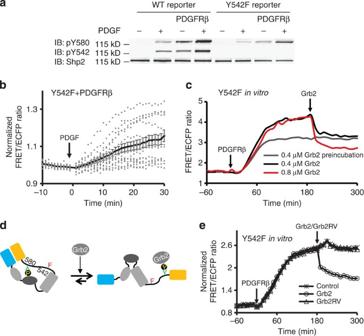Figure 4: Grb2 cantrans-interact with Shp2. (a) The phosphorylation of WT and Y542F reporters before and after 5 min PDGF stimulation in MEFs with or without the overexpression of PDGFRβ. (b) The ratio time courses of Y542F reporter before and after PDGF stimulation in MEFs overexpressing PDGFRβ. The dotted lines from each cell are overlaid with the solid curve (mean±s.e.m.). (c) The PDGFRβ-induced ratio changes of Y542F reporter pre- or post-incubated with Grb2in vitro. (d) The model depicts the effect of Grb2 in altering the Y542F reporter conformations. (e) The ratio time courses of the Y542F reporterin vitroupon PDGFRβ incubation, followed by the addition of Grb2 or Grb2RV. Figure 4: Grb2 can trans -interact with Shp2. ( a ) The phosphorylation of WT and Y542F reporters before and after 5 min PDGF stimulation in MEFs with or without the overexpression of PDGFRβ. ( b ) The ratio time courses of Y542F reporter before and after PDGF stimulation in MEFs overexpressing PDGFRβ. The dotted lines from each cell are overlaid with the solid curve (mean±s.e.m.). ( c ) The PDGFRβ-induced ratio changes of Y542F reporter pre- or post-incubated with Grb2 in vitro . ( d ) The model depicts the effect of Grb2 in altering the Y542F reporter conformations. ( e ) The ratio time courses of the Y542F reporter in vitro upon PDGFRβ incubation, followed by the addition of Grb2 or Grb2RV. 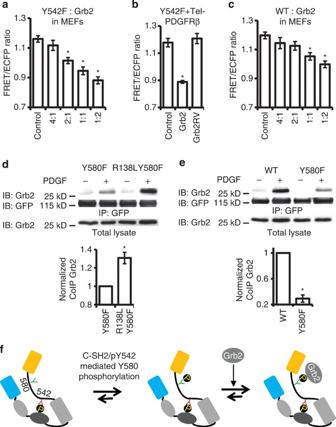Figure 5: Grb2 tunes thecis-interaction of Shp2 in MEFs. (a–c) The averaged ratios of the Y542F (a,b) or WT (c) reporter in MEFs coexpressing Tel-PDGFRβ with control vector, different amounts of Grb2 (a,c), or Grb2RV (b). (a)n=16, 17, 14, 18, 11, *,P<4.55e−5; (b)n=38, 25, 26, *,P<1.0e−8; (c)n=10, 20, 18, 15, 35, *P<3.1e−4 (Student’st-test with Bonferroni correction). (d–e) The amount of Grb2 coimmunoprecipitated with WT or its mutant reporters in MEFs before and after 15 min PDGF stimulation. *,P<0.05 (Student’st-test,n=3). Bar graphs represent the mean±s.e.m. of normalized intensity against its corresponding control group (refer toSupplementary Fig. S7afor the whole blots). (f) The model depicts the early interaction of C-SH2/pY542, the subsequent pY580 phosphorylation which recruits Grb2 and is sequestered by Grb2 to stabilize this C-SH2/pY542 pair. Full size image Figure 5: Grb2 tunes the cis -interaction of Shp2 in MEFs. ( a – c ) The averaged ratios of the Y542F ( a,b ) or WT ( c ) reporter in MEFs coexpressing Tel-PDGFRβ with control vector, different amounts of Grb2 ( a,c ), or Grb2RV ( b ). ( a ) n =16, 17, 14, 18, 11, *, P <4.55e−5; ( b ) n =38, 25, 26, *, P <1.0e−8; ( c ) n =10, 20, 18, 15, 35, * P <3.1e−4 (Student’s t -test with Bonferroni correction). ( d – e ) The amount of Grb2 coimmunoprecipitated with WT or its mutant reporters in MEFs before and after 15 min PDGF stimulation. *, P <0.05 (Student’s t -test, n =3). Bar graphs represent the mean±s.e.m. of normalized intensity against its corresponding control group (refer to Supplementary Fig. S7a for the whole blots). ( f ) The model depicts the early interaction of C-SH2/pY542, the subsequent pY580 phosphorylation which recruits Grb2 and is sequestered by Grb2 to stabilize this C-SH2/pY542 pair. Full size image Rewired Shp2 reprograms cis -interaction and ERK dynamics Based on the results, it is clear that the Y542 contextual sequence is favoured as a substrate for PDGFR and has a higher affinity for C-SH2 upon phosphorylation. However, position 580 is favoured by C-SH2 for the cis -interaction over position 542 within the context of the intact Shp2 molecule. This antagonistic combination of sequence and position results in a favoured cis -interaction between C-SH2 and Y580 in vitro , where both Y542 and Y580 are independently phosphorylated by the PDGFR in solution. In MEFs, the recruitment of Shp2 to the membrane receptor PDGFR through its N-SH2 domain [25] leads to an early phosphorylation of the favoured substrate Y542, which subsequently undergoes cis -interaction with C-SH2. This pY542/C-SH2 interaction and the resulted conformational change are essential and facilitate the phosphorylation of Y580, which recruits Grb2 to sequester the otherwise favoured pY580 from competing for the pY542-occupied C-SH2. As such, Grb2 in MEFs can bind to pY580 and shift the equilibrium of cis -interaction towards pY542/C-SH2, distinct from the dominant pY580/C-SH2 cis -interaction of Shp2 in solutions. It hence becomes apparent that the moderate difference between pY542 and pY580 in competing for C-SH2, resulting from the antagonistic combination of tyrosine sequence and position, can allow easier alteration of Shp2 cis -interactions by Grb2 binding. We have then rewired the modular arrangement within Shp2 to develop a SWAP reporter by swapping the Y542 and Y580 sequences to combine the favourable Y542 sequence with the preferred 580 position in a synergistic fashion (Y542’: Y580 sequence at 542 position; Y580’: Y542 sequence at 580 position), widening the gap of competitiveness between the two tyrosines ( Fig. 6a ). 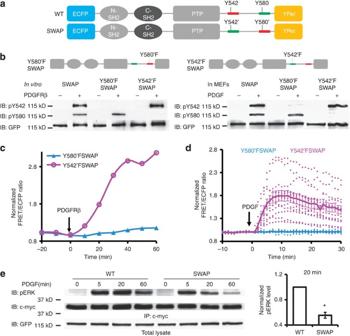Figure 6: The loss of tunablecis-interaction within the SWAP reporter and its effect on ERK phosphorylation. (a) Schematic drawings and comparison of the WT and SWAP Shp2 reporters. Y542 and Y580 sequences are coloured in red and green, respectively. (b) The phosphorylation of SWAP and its mutant reportersin vitro(left) or in MEFs (right, whole-cell lysate). (c,d) The ratio changes of Y542’FSWAP and Y580’FSWAP reporters (c)in vitroor (d) in MEFs. (e) The ERK phosphorylation at different time points (left) and its quantification (mean±s.e.m.) at 20 min (right) upon PDGF stimulation in MEFs expressing either WT or SWAP reporter as indicated. *,P<0.05 (Student’st-test,n=3, refer toSupplementary Fig. S7bfor the whole blots). Figure 6: The loss of tunable cis -interaction within the SWAP reporter and its effect on ERK phosphorylation. ( a ) Schematic drawings and comparison of the WT and SWAP Shp2 reporters. Y542 and Y580 sequences are coloured in red and green, respectively. ( b ) The phosphorylation of SWAP and its mutant reporters in vitro (left) or in MEFs (right, whole-cell lysate). ( c,d ) The ratio changes of Y542’FSWAP and Y580’FSWAP reporters ( c ) in vitro or ( d ) in MEFs. ( e ) The ERK phosphorylation at different time points (left) and its quantification (mean±s.e.m.) at 20 min (right) upon PDGF stimulation in MEFs expressing either WT or SWAP reporter as indicated. *, P <0.05 (Student’s t -test, n =3, refer to Supplementary Fig. S7b for the whole blots). Full size image We thereafter examined the characteristics of the SWAP reporter in vitro and in MEFs. Y542’ and Y580’ of the SWAP reporter were phosphorylated independently both in vitro and in MEFs ( Fig. 6b ). PDGF also induced a remarkably high FRET change of the SWAP reporter in MEFs, significantly stronger than that of the WT reporter and with a level as high as the in vitro response ( Supplementary Fig. S4a,b ; Fig. 3b , Supplementary Movie 4 ). More importantly, Y580’F or R138L, but not Y542’F nor R32L, abolished the FRET response of the SWAP reporter both in vitro and in MEFs ( Fig. 6c ; Supplementary Fig. S4c,d ; Supplementary Movie 5 and 6 ). These results confirmed that the SWAP reporter loses the tunable cis -interactions with its C-SH2 undergoing one form of cis -interaction with the pY580’ both in vitro and in MEFs. The Y542’ phosphorylation of SWAP reporter was also lower than that of WT reporter ( Supplementary Fig. S4e ), suggesting that the regulatory mechanism of promoting Y580 phosphorylation by C-SH2/pY542 cis -interaction no longer exists in the SWAP reporter. Consequently, this rewired cis -regulation of Shp2 conformation caused a significantly more transient ERK phosphorylation upon PDGF stimulation ( Fig. 6e , Supplementary Fig. S4f ). Therefore, by swapping the Y542 and Y580 sequences, we have rewired the regulation mechanism of Shp2 conformation, which led to a reprogrammed downstream ERK signalling. Our results indicate that a simple antagonistic combination of contextual sequence and position can result in tunable cis -interactions within Shp2, leading to complex regulation routes and functional outcomes. pY542 in the WT reporter has the combination of favoured sequence and adverse position while pY580 has adverse sequence and favoured position. Swapping the sequences results in a synergistic combination: pY580’ with favoured sequence and position while pY542’ with adverse sequence and position ( Fig. 6a ). As such, the order of these four phosphotyrosines in terms of their affinity for C-SH2 is as follows: pY542’<pY542<pY580<pY580’. Therefore, the antagonistic combination has two layers of effect on the cis -interactions of Shp2. First, it ensures that the affinity of both pY542 and pY580 in WT Shp2 for cis -regulation is moderate enough to allow effective trans -regulations and prevent possibly insurmountable cis -interactions as in the case of pY580’. This note is supported by the observation that Grb2 more effectively inhibit the FRET response of Y542 reporter (pY580 and C-SH2 cis -interaction) than that of Y542’FSWAP (pY580’ and C-SH2 cis -interaction) ( Supplementary Fig. S5a ). In addition, the affinity of Grb2 towards isolated pY542 or pY580 peptide is several orders higher than that of C-SH2 ( Table 1 ). This higher affinity of Grb2 allows the effective competitiveness of trans -interaction, overcoming the entropic advantage of cis -interactions within the WT Shp2 (ref. 26 ). Second, the antagonistic combination can lead to a relatively small difference in the cis -interaction competitiveness between the two phosphotyrosines than the synergistic combination (pY580–pY542<pY580’–pY542’). Therefore, the presence of Grb2 in mammalian cells can tune the cis -interaction of WT Shp2 towards pY542/C-SH2 pair from pY580/C-SH2 pair. In contrast, the pY580’/C-SH2 pair in SWAP reporter dominates both in cells and in vitro . As such, the synergistic combination in the SWAP reporter resulted in the enlargement of the difference in competitiveness between the two phosphotyrosines, the inhibition of Grb2-mediated trans -regulation, the loss of tunable cis -interactions within Shp2 and eventually the reprogramming of downstream ERK signalling dynamics. This combinatorial effect of protein modules is strikingly similar to that of DNA cis -regulatory elements on regulating a coordinated gene expression where sequence-specific promoters/enhancers are highly structured and precisely positioned [4] , [5] , [27] . We suggest that this antagonistic combination of protein sequence and position can serve as a basic design principle for the construction of tunable protein elements and building blocks to develop higher order and programmable molecular machineries, capable of learning and adapting according to environmental cues. Systems and synthetic biologists have long employed networks to describe the signalling transduction, with each node representing one molecule and its determined function [28] . We discovered in this work that a tunable regulation mechanism is embedded within one molecule, for the processing of environmental inputs to result in differential Shp2 conformations and functional outcomes. These cis -interactions within Shp2 allow the fine regulation of protein functions beyond the simple disruption of autoinhibition for protein activations. This protein-based regulation can also produce fast responses at specific subcellular locations, surpassing the capacity of gene-based tuning of cellular functions [29] . Hence, this tunable regulation mechanism built in Shp2 may provide a prominent example on how nature can design/evolve molecules with their conformations/functions differentially regulated under different subcellular environments. Integrating with molecular switches/gates based on scaffold proteins [30] , [31] and genetic circuits [29] , the understanding and rewiring of these modular motif arrangements may also provide powerful means to reprogram the downstream signalling cascades at subcellular levels [28] . It is of note that the tunable cis -interactions within Shp2 may not exist in lower organisms as the Drosophila ortholog, Corkscrew, only retains Y542 while the Caenorhabditis elegans ortholog, Ptp-2, lacks both tyrosines [18] . Therefore, this cis -regulatory mechanism of Shp2 may represent a distinguished evolutionary innovation in higher organisms for the fine-tuning of functions resulting in higher levels of organism complexity [32] . In addition, our results show that Grb2 can tune the cis -interaction of Shp2. However, Grb2 may not be the only molecule that can trans -regulate Shp2 function, as Grb2 short interfering RNA (siRNA) knockdown did not increase the FRET level of Y542F reporter compared with control siRNA ( Supplementary Fig. S5b ). Our FRET-based Shp2 reporter mainly revealed the cis -interactions between phosphotyrosines and C-SH2, but not N-SH2. It appears unlikely that N-SH2 has cis -interactions with pY542 or pY580 as the binding cleft of N-SH2 domain in the full-length Shp2 is in a compressed and closed conformation limiting accessibility for phosphopeptides [33] , [34] . It has been established that the phosphotyrosine interaction of N-SH2 can drastically affect the Shp2 phosphatase activity by relieving the autoinhibitory cis -interaction between N-SH2 and PTP domain [35] , [36] . In our study, the binding of C-SH2 by either pY542 or pY580 did not have significant impact on the phosphatase activity as the phosphatase activity of R32L reporter did not increase after being phosphorylated by PDGFR kinase ( Supplementary Fig. S5c,d ). Therefore, the SH2 domain interactions within Shp2 can have two main functional outcomes: the trans -interaction of N-SH2 regulates enzymatic phosphatase activity, whereas that cis -interaction of C-SH2 controls the Y580 phosphorylation and the subsequent Grb2 recruitment to govern downstream signalling cascades, such as ERK phosphorylation. While the initial phosphorylation of ERK is mainly dependent on the receptor-Ras pathway [37] , the phosphorylation of Y580 is crucial for the maintenance of a sustained ERK phosphorylation [22] . Indeed, it has been proposed that pY580 may serve as a docking site for Grb2/Sos complex and, therefore, regulate downstream ERK pathway [38] . In the SWAP reporter, pY542’ was also constitutively lower ( Supplementary Fig. S4e ), causing a transient ERK phosphorylation ( Fig. 6e ). As the different dynamics of ERK activation has been shown to determine cell fate and long-term memory [39] , [40] , the wiring and rewiring of Y542 and Y580 positions in Shp2 to control pY580/pY542’ and hence ERK phosphorylation dynamics can have profound impact on pathophysiological consequences. The modular SH2-phosphotyrosine trans -interaction between different proteins has been well established to mediate molecular interactions and signalling transduction [41] . The intramolecular cis -interaction of SH2-phosphotyrosine has also been shown to regulate the molecular functions [42] . For example, the cis -interaction between pY527 and SH2 domain of Src kinase can cause the autoinhibition of Src kinase domain [43] . The SH2-phosphotyrosine trans -interaction can further compete for the cis -interaction of domains within a molecule and modulate the molecular function. Indeed, Src SH2 domain can interact with pY397 at FAK to release the FERM domain from masking the FAK kinase domain and cause FAK activation [44] . However, most studies involve only one pair of SH2-phosphotyrosine interaction. The Shp2 molecule has two coordinating pairs of SH2-phosphotyrosine interaction. Our results suggest that an antagonistic combination of sequence and position of the phosphorylated tyrosines can result in tunable cis -interactions within one molecule to allow effective trans -regulations of its conformational changes and subsequently functions. With the prevalence of SH2-phosphotyrosine and other modules, the complexity of cis -interactions between multiple interacting domains revealed by our FRET-based study may be a typical but overlooked layer that contributes to the overall complexity of cell signalling. Reporter construction and other constructs The Shp2 reporter was constructed by fusing a full-length human Shp2 complementary DNA to an N-terminal ECFP sequence and a C-terminal YPet sequence in pRSETb (Invitrogen) for bacterial expression. For mammalian cell expression, the Shp2 reporter was cloned into pcDNA3.1 (Invitrogen) behind a Kozak sequence using Bam HI/ Eco RI restriction sites. Point mutations of the Shp2 reporters were generated using QuikChange Site-Directed Mutagenesis Kit (Agilent Technologies). Deletion or insertion mutations of Shp2 reporter were generated by PCR and subsequent ligation. The sequence of 11 aa(s) surrounding Y542 or Y580 (including four residues in front of and six residues behind tyrosine) was referred as Y542 or Y580 sequence, respectively. The Δ542 reporter has a truncation between residue 538 and 575, whereas the Δ580 reporter has a truncation between residue 556 and 593. The SWAP reporter has the 11 aa sequences surrounding Y542 and Y580 exchanged. The Y542Y542 reporter has the Y542 sequence at both Y542 and Y580 positions. Tel-PDGFRβ constructs were from Dr Gary Gilliland. Protein expression and purification HEK cells (ATCC) transfected with WT or mutated Shp2 reporters were washed with cold PBS and then lysed in buffer containing 50 mM Tris–HCl pH 7.5, 100 mM NaCl, 1 mM EDTA, 0.2 mM phenylmethylsulphonyl fluoride, 0.2% Triton X-100 and a protease inhibitor cocktail tablet (Roche). Lysates were centrifuged at 10,000 g at 4 °C for 10 min. Supernatants were incubated with Ni-NTA agarose beads (Qiagen), which were then washed with 50 mM Tris–HCl pH 7.5, 100 mM NaCl, 10 mM imidazole. Reporter proteins were eluted in a buffer containing 50 mM Tris–HCl pH 7.5, 100 mM NaCl and 100 mM imidazole. Alternatively, reporter proteins were purified from E. coli for large quantities. Reporters in pRSETb were transformed into BL21 and the expression was induced by exposure to 0.4 mM isopropyl-β- D -thiogalactoside for 16 h at room temperature (RT). The bacteria were lysed in buffer A (20 mM imidazole, 20 mM Tris–HCl pH 8, 200 mM NaCl) with EmulsiFelx-B15 (Avestin). Lysates were centrifuged at 10,000 g at 4 °C for 20 min. Supernatants were then loaded onto a HisTrap HP column using an AKTA purifier FPLC system (GE). The column was subsequently washed with 20 ml of buffer A and the fusion protein eluted using a 20–400 mM imidazole concentration gradient developed in 50 ml buffer A at 0.5 ml min −1 . Fractions with absorption at 430 nm were pooled, concentrated and subsequently loaded onto a HiLoad 16/60 Superdex 200 gel filtration column (GE). Buffer B (30 mM Tris-HCl pH 8.0, 200 mM NaCl, 1 mM dithiothreitol) was then used for elution. Fractions around molecular weight 120 kDa were collected and concentrated for in vitro assays. Immunoprecipitation and immunoblotting Cells were washed three times with ice-cold PBS and lysed in a buffer (Cell Signaling) containing 50 mM Tris–HCl, pH 7.5, 125 mM NaCl, 1% Triton X-100, 0.1% SDS, 5 mM NaF, 1 mM Na 3 VO 4 , 1 mM phenylmethylsulfonyl fluoride and 10 μg ml −1 leupeptin. Lysates were centrifuged at 10,000 g at 4 °C for 10 min, and the protein concentration of clarified lysates was determined by Bradford assay (Biorad). Antibodies (1 μg per 100 μg total lysate) for Co-immunoprecipitation (IP) or IP were incubated with cell lysates for 1 h at 4 °C. Protein A/G beads (Santa Cruz) were then added to the mixture and incubated overnight at 4 °C. The beads were washed three times with lysis buffer and boiled for 5 min in SDS protein loading buffer. After centrifugation, the supernatants were resolved by SDS–polyacrylamide gel electrophoresis. The proteins were then transferred onto a nitrocellulose membrane and blocked with 5% bovine serum albumin in TTBS buffer (50 mM Tris–HCl, 145 mM NaCl, 0.05% Tween-20, pH 7.4) for 2 h at RT. Membranes were further incubated with primary antibodies overnight at 4 o C, washed and then incubated with horseradish peroxidase-conjugated secondary antibodies for 2 h at RT. Signals were detected using SuperSignal Western Pico or Femto ECL Kit (Pierce). Western results were quantified with ImageJ (NIH). Our statistics were performed with two-tailed Student’s t -test. When multiple t -tests were performed, the α-value was modified by the Bonferroni correction, such that α =0.0125 for up to four t -tests performed in each group ( Fig. 5 ). Anti-phospho-SHP-2 (Tyr-542) and (Tyr-580) antibodies were from Cell Signaling Technology (Cat # 3751 and 3703). Anti-GFP antibody for IP was from Abcam (Cat # ab290). Anti-phosphotyrosine pY20 antibody was from BD Transduction laboratory (Cat # 610000). Anti-Shp2, anti-GFP antibodies for immunoblotting, as well as HRP-conjugated secondary antibodies were purchased from Santa Cruz Biotechnology (Cat # sc-280, sc-8334, sc-2004, sc-2005). Image acquisition and analysis Glass-bottom dishes (Cell E&G Inc.) were coated with 10 μg ml −1 fibronectin (Sigma) overnight at 37 °C. Transfected MEFs were plated onto these dishes overnight in DMEM containing 0.5% FBS before imaging. During imaging, MEFs (ATCC) were maintained in CO 2 -independent medium (Invitrogen) with 0.5% FBS at 37 °C for 10 min before treatment with 20 ng ml −1 PDGF (Sigma). Images were obtained on a Zeiss Axiovert inverted microscope equipped with a cooled charge-coupled device camera (Cascade 512B; Photometrics) using MetaFluor 6.2 software (Molecular Devices). The following filter sets (Chroma) were used in our experiments for FRET imaging: a dichroic mirror (450 nm), an excitation filter 420/20 nm, an ECFP emission filter 475/40 nm, and a FRET emission filter 535/25 nm. The excitation filter for ECFP at 420±20 nm was specifically selected to shift towards lower wavelength away from the peak excitation spectrum of ECFP to reduce the cross-excitation of the FRET acceptor YPet, which has significantly higher brightness than ECFP. This filter selection can minimize the effect of bleed-through on the FRET channel. The fluorescence intensity of non-transfected cells was quantified as the background signal and subtracted from the ECFP and FRET signals of transfected cells. The pixel-by-pixel ratio images of FRET/ECFP were calculated based on the background-subtracted fluorescence intensity images of ECFP and FRET by using the MetaFluor software. These ratio images were displayed in the intensity modified display mode in which the colour and brightness of each pixel is determined by the FRET/ECFP ratio and ECFP intensity, respectively. The emission ratio were quantified and analysed by Excel (Microsoft). In vitro kinase assays Purified proteins were dialyzed overnight at 4 °C in kinase buffer (50 mM Tris–HCl pH 8.0, 100 mM NaCl, 10 mM MgCl 2 and 2 mM dithiothreitol). Fluorescence emission spectra of the purified reporters (0.5 μM) were measured in 96-well plates with an excitation wavelength of 430 nm using a fluorescence plate reader (TECAN, Sapphire II). Emission ratios of acceptor/donor (526 nm/478 nm) were measured at 30 °C before and after the addition of 1 mM ATP and 10–100 nM active PDGFRβ kinases (Millipore). Affinity measurement by SPR The binding affinity of pY542 and pY580 peptides to C-SH2 domain or Grb2 was assessed by SPR analysis on a BIAcore 3000 instrument (GE). Biotinylated peptides were immobilized on streptavidin-coated SA sensor chips (GE). Before immobilization, the sensor chip was conditioned with a solution containing 1 M NaCl and 50 mM NaOH. The binding assays were conducted at RT in HBS-EP buffer (GE, 10 mM HEPES, pH 7.4, 150 mM NaCl, 3 mM EDTA, 0.005% Surfactant P20). Each pY peptide was injected at a flow rate of 5 μl min −1 until a constant level of response units (500–600 RU) was obtained. Varying concentrations of histidine-tagged C-SH2 or Grb2 were passed over the immobilized peptides for 2 min. To remove the proteins from the peptide, a regeneration buffer (10 mM NaOH, 200 mM NaCl, 0.05% SDS) was applied. The equilibrium response unit (RU eq ) at a given protein concentration was obtained by subtracting the response of a blank control chip. The dissociation constants ( K d ) were calculated by the BIAevaluation software using the equation 1, where RU eq is the measured response unit at a given SH2 domain concentration, and RU max is the maximum response unit: Immunostaining Cells were washed three times with ice-cold PBS and fixed with 4% paraformaldehyde at RT for 15 min before they were permeabilized with 0.1% TritonX-100 in PBS for 30 min. After that, the cells were rinsed and blocked with 1% BSA in PBS for 20 min. They were then incubated with primary antibody (Santa Cruz, Cat # sc-280 or sc-8994, 1:1,000 dilution) in PBS at RT for 2 h before they were incubated with secondary antibody conjugated with fluorescence dye at RT for 1 h. After another round of washing, the cells were subjected to imaging under microscopy. Phosphatase activity assays Phosphatase activity was measured using fluorogenic 6,8-difluoro-4-methylumbelliferyl phosphate (DiFMUP; Invitrogen) as the substrate. Each reaction contained 50 mM Tris pH 8, 100 mM NaCl, 10 mM MgCl 2 , 2mM dithiothreitol, 20 μM DiFMUP and 20 nM Shp2 reporter in a total reaction volume of 100 μl in a well of 96-well plates. Reactions were initiated by the addition of DiFMUP, followed by incubation for 30 min at 30 o C. The fluorescence signal of the reaction product, 6,8-difluoro-4-methylumbelliferone, was measured at an excitation wavelength of 355 nm and an emission of 460 nm with a plate reader. How to cite this article: Sun, J. et al . Antagonism between binding site affinity and conformational dynamics tunes alternative cis -interactions within Shp2. Nat. Commun. 4:2037 doi: 10.1038/ncomms3037 (2013).